Poly-cyclodextrin and poly-paclitaxel nano-assembly for anticancer therapy Effective anticancer therapy can be achieved by designing a targeted drug-delivery system with high stability during circulation and efficient uptake by the target tumour cancer cells. We report here a novel nano-assembled drug-delivery system, formed by multivalent host–guest interactions between a polymer–cyclodextrin conjugate and a polymer–paclitaxel conjugate. The multivalent inclusion complexes confer high stability to the nano-assembly, which efficiently delivers paclitaxel into the targeted cancer cells via both passive and active targeting mechanisms. The ester linkages between paclitaxel and the polymer backbone permit efficient release of paclitaxel within the cell by degradation. This novel targeted nano-assembly exhibits significant antitumour activity in a mouse tumour model. The strategy established in this study also provides knowledge for the development of advanced anticancer drug delivery. Drug-loaded polymeric nanocarriers are of immense interest as anticancer drug-delivery systems due to their ability to extravasate within the tumours via the enhanced permeation and retention (EPR) effect [1] , [2] , [3] , [4] . Polymeric delivery systems can also enhance the aqueous solubility and modify the pharmacokinetics and biodistribution of lipophilic drugs [5] , [6] , [7] , [8] , [9] , [10] , [11] , [12] . However, not all polymeric nanocarriers work efficiently. For example, some polymeric micelles formed via self-assembly of amphiphilic block copolymers are unstable when diluted below their critical micelle concentration within the circulatory system; this can result in a burst release of drugs that may cause significant toxicity to healthy cells. Although polymer–drug conjugates minimize such an initial burst of drug and may also enhance the solubility of hydrophobic drugs, they still may be less effective than a free drug when taken up into cells due to imperfect degradable characteristics of polymer–drug conjugates [8] , [9] , [10] , [11] . To maximize the efficacy of drugs, the conjugated drugs should undergo intracellular enzyme-mediated release in their free forms after entering the cells. Therefore, an efficient drug delivery should provide stability of the delivery system during circulation and rapid enzymatic degradation of the drug carrier after cellular uptake. For efficient cellular uptake, it is also highly essential to conjugate cell-specific targeting ligands to the carriers. These ligand-conjugated carriers with improved stability may increase the blood circulation time and frequency of encounter with the target cells, which eventually allows the carriers to recognize, bind and internalize efficiently in the cells through a receptor-mediated endocytosis process. It is well known that cyclodextrin (CD) can form inclusion complexes with various hydrophobic drugs [13] , [14] , [15] , [16] , [17] . It is also well known that paclitaxel (PTX), one of the most common antitumour drugs [18] , [19] , [20] , forms an inclusion complex with beta-CD (β-CD), which results in a significant increase in the aqueous solubility of PTX [21] , [22] , [23] , [24] , [25] , [26] . Therefore, it is to be expected that multivalent inclusion complexes will form between two functionalized polymers with multiple CDs and multiple PTXs attached to each of the polymer backbones, respectively. It is also expected that such multivalent polymer–polymer complexations will yield a strong nano-assembly. In addition, it is important to note that the drug PTX must be easily released from this novel nano-assembly, and this can be promoted by using degradable ester linkages between PTX and corresponding polymer. Applying these rational design principles, we report here a novel nano-assembly composed of polymeric CD (pCD) and polymeric PTX (pPTX), with the CD and PTX molecules each being linked to the polymer backbone by degradable ester groups. The polymer backbones are copolymers of maleic anhydride (MAnh), which reacts with hydroxyl groups of CD or PTX to open up and form CD or PTX ester linkages and carboxylate groups. The pPTX/pCD nano-assembly not only shows good water dispersibility due to the negative carboxylate ions on both pCD and pPTX, but also exhibits high stability in the blood due to the multivalent host–guest interactions. The nano-assembly is efficiently taken up by the targeted cancer cells via passive and active targeting mechanisms, and releases PTX from the nano-assembly by intracellular esterase, and thereby effectively demonstrates a long-term in vivo antitumour effect. This novel strategy may provide future directions for designing an effective anticancer drug-delivery system with enhanced stability in the circulatory system, tumour-targeted delivery and intracellular drug release. Rational design of a nano-assembly The delivery system is composed of a stable, water-dispersible, nano-assembled particle formed from the inclusion complexation of a polymer-CD (pCD) conjugate and a polymer-PTX (pPTX) conjugate. The CD and PTX molecules are conjugated via their OH groups to a MAnh copolymer backbone to form enzyme-degradable and hydrolyzable ester linkages to the polymers ( Fig. 1 ). It is important to note that each time a CD or PTX is conjugated by an ester linkage to an anhydride moiety of the polymer, a carboxylate ion is also formed, and these groups will significantly enhance the water dispersibility of the nano-assembly being formed. Since PTX is not only conjugated to a polymer chain but also complexed within a CD that is conjugated to another polymer, the loading of the PTX drug into the nano-assembly can be significantly increased. Furthermore, this nano-assembly can maintain its structural integrity even in low concentrations due to multivalent interactions between the CD- and PTX-conjugated polymers. 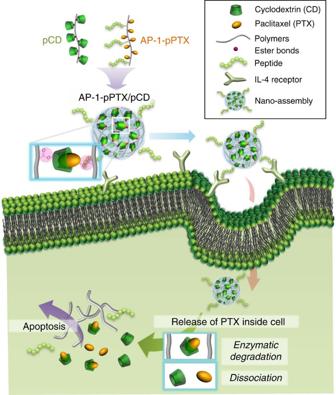Figure 1: Schematic representation of nano-assembly-mediated PTX delivery. The nano-assembly is formed by multivalent inclusion complexes between pCD and pPTX. It exhibits high stability during blood circulation due to the multivalent host–guest interaction. After the nano-assembly is delivered into the targeted cancer cells via passive and active targeting mechanism, drug is efficiently released from the nano-assembly by the enzymatic degradation and induces the apoptosis of cancer cells. Figure 1: Schematic representation of nano-assembly-mediated PTX delivery. The nano-assembly is formed by multivalent inclusion complexes between pCD and pPTX. It exhibits high stability during blood circulation due to the multivalent host–guest interaction. After the nano-assembly is delivered into the targeted cancer cells via passive and active targeting mechanism, drug is efficiently released from the nano-assembly by the enzymatic degradation and induces the apoptosis of cancer cells. Full size image Preparation of the pPTX/pCD nano-assembly We used two copolymers of MAnh as backbone polymers: poly(isobutylene- alt -MAnh) (poly[IB- alt -MAnh], molecular weight (Mw) 6 kDa) and poly(methyl vinyl ether- alt -MAnh) (poly[MVE- alt -MAnh], Mw 80 kDa). The copolymers of MAnh are considered to be versatile reactive and functional polymers, which can be readily obtained through copolymerization of MAnh with other suitable olefin monomers. Further, the reactive anhydride moiety in the backbone of the MAnh copolymer allows facile conjugation with a wide range of therapeutic drugs under mild reaction conditions. The macromolecular–drug conjugates produced using MAnh copolymers have demonstrated excellent pharmacological properties compared with free drugs. In this study, poly[IB- alt -MAnh] was chosen because of its low Mw for easy renal clearance, while poly[MVE- alt -MAnh] was chosen because of its greater water solubility, which is needed for conjugating to the highly hydrophobic PTX. pCD and pPTX were synthesized by conjugation of CD and PTX into poly[IB- alt -MAnh] and poly[MVE- alt -MAnh], respectively ( Fig. 2a ). The details of synthesis are described in the Method section. 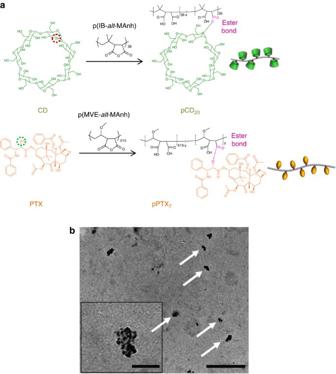Figure 2: Synthesis and characterization of pCD and pPTX. (a) Synthetic scheme of pCD and pPTX conjugate. Each hydroxyl group of CD (red circle) and PTX (green circle) was activated by LiH and sequentially conjugated to each poly(MAnh). (b) TEM image of the pPTX/pCD nano-assembly (scale bar, 500 nm). Each white arrow indicates the individual pPTX/pCD nano-assembly. Inset is a magnified image (scale bar, 100 nm). Figure 2: Synthesis and characterization of pCD and pPTX. ( a ) Synthetic scheme of pCD and pPTX conjugate. Each hydroxyl group of CD (red circle) and PTX (green circle) was activated by LiH and sequentially conjugated to each poly(MAnh). ( b ) TEM image of the pPTX/pCD nano-assembly (scale bar, 500 nm). Each white arrow indicates the individual pPTX/pCD nano-assembly. Inset is a magnified image (scale bar, 100 nm). Full size image During the dialysis purification process, the unreacted anhydride groups of the CD- and PTX-conjugated copolymers were converted to carboxylic acid groups, resulting in water-soluble polymer conjugates. The conjugation ratios of pCDs and pPTXs were characterized by 1 H-NMR ( Supplementary Figs 1 and 2 ), and the results are listed in Supplementary Table 1 . In 1 H-NMR, the chemical conjugation between CD and poly[IB- alt -MAnh] was confirmed by the reduced integration value of the hydroxyl group at the 2-position of CD and an increased integration value at 4.2–4.6 p.p.m., which indicates the summation of the hydroxyl group at the 6-position and the proton at the ester-formed 2-position in pCD ( Supplementary Fig. 1 ). The hydroxyl group of the 2′-position disappeared, and the proton of the 2′-position was up-shifted in the 1 H-NMR of pPTX, indicating the successful formation of an ester bond between PTX and poly[MVE- alt -MAnh] ( Supplementary Fig. 2 ). Among the combinations of pCD and pPTX conjugates, pCD 20 and pPTX 7 were used for further study due to their enhanced water solubility. The pPTX/pCD (molar ratio of PTX/CD=1:1) nano-assembly was formulated by dissolving the two polymer conjugates in a water–ethanol solution, followed by freeze drying. To verify the formation of the polymeric nano-assembly and to determine its size, we used dynamic light scattering (DLS) and transmission electron microscopy (TEM). The average radius of the nano-assembly in water was 54.6±11.6 nm ( Supplementary Table 2 ). Compared with aqueous dispersions of pPTX or pCD, this nano-assembly had a very small size and a narrow size distribution ( Supplementary Fig. 3 ), confirming the successful fabrication of the nano-assembly. As shown in Fig. 2b , the TEM image revealed that the nano-assembly comprised small ellipsoidal particles. The pPTX/pCD nano-assembly may reach a limiting size (for example, radius, around 50 nm) as a result of the appropriate balance of two interconflicting traits, namely, continuous formation of polymeric inclusion complexes and increasing repulsion of carboxylate ions within the polymer backbones. Stability and solubility of the pPTX/pCD nano-assembly Because of the multiple interactions, it is expected that the nano-assembly formed via a multivalent inclusion complex between pCD and pPTX can show higher stability than that of the monovalent PTX/CD. Therefore, to demonstrate the robustness of this nano-assembly, the association constant ( K a ) of pPTX/pCD was experimentally determined by the competition reaction with 6-( p -toluidino-2-naphthalenesulfonic acid) (TNS), which is known to bind strongly to CDs [27] , [28] . 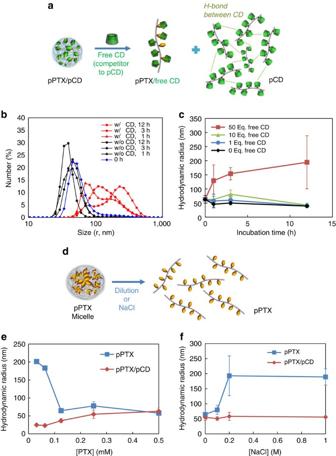Figure 3: Stability study of the pPTX/pCD nano-assembly and pPTX micelle. (a) Illustration of the dissociation of the pPTX/pCD complex in the presence of free CD. (b) The change in hydrodynamic radius distribution of the pPTX/pCD complex by adding 50 equivalent free CD. (c) The hydrodynamic radius profiles of pPTX/pCD during incubation with various equivalents free CD. (d) Illustration of pPTX micelle disruption by dilution or NaCl addition. (e) The effect of [PTX] concentration (based on the amount of PTX in pPTX) on the size of the pPTX/pCD and the pPTX micelle, as [PTX] increases from 0.03 to 0.5 mM. (f) The salt effect on the size of pPTX/pCD and pPTX micelle, where [PTX]=0.125 mM, [NaCl]=0, 0.1, 0.2 and 1.0 M. Error bars represent ±s.d. fromn=3. The pPTX/pCD nano-assembly has a 10 4 -fold higher K a value compared with the monovalent complex PTX/CD ( Supplementary Table 3 and Supplementary Fig. 4 ). The nano-assembly can be disrupted into small subparticles by adding excess free CD, because it will compete with pCD in forming the inclusion complex. Therefore, the size change of the nano-assembly was investigated after the addition of excess free CD. When free CD (50 equivalent per PTX/CD moiety in nanoparticle (NP)) was added to the nano-assembly, a rapid increase in size up to several hundred nm and a substantial change in the size distribution was observed; meanwhile pPTX/pCD remained stable for 12 h in PBS ( Fig. 3a–c ). This result suggests the pPTX/pCD network is disrupted due to the insertion of free CD into the nano-assembly between pPTX and pCD, forming an uncomplexed pCD group and a pendant pPTX molecule complexed to the free CD. This observation provides further evidence that the small and dense pPTX/pCD nano-assembly was formed by many host–guest interactions between pPTX and pCD. Noticeably, concentrations less than 50 equivalent of free CD did not induce any size enhancement of the pPTX/pCD ( Fig. 3c ), suggesting that the nano-assembly is stable and resistant to disruption. Thus, this nano-assembly can act as a circulating ‘depot’ of PTX that is ready to be entrapped in tumour tissue by the EPR effect. Considering the propensity of polymeric micelles to undergo dissociation under the high dilution and salt concentration occurring during intravenous administration, we also evaluated the effect of the concentration of PTX in pPTX micelles and ionic strength on the size of the pPTX/pCD nano-assembly [29] . As shown in Fig. 3d–f , the size of pPTX/pCD was not strongly influenced by the PTX concentration or by the salt concentration, indicating robustness of the pPTX/pCD nano-assembly. In contrast, pPTX micelles were destabilized at a low concentration of the PTX micelles and at a high salt concentration. It is possible that 0.1 mM pPTX might be lower than the critical micelle concentration of pPTX, which easily disassociated the pPTX micelles. Also, the high concentration of NaCl would compress the double layer and neutralize the surface charge of pPTX micelles, which removes the electrostatic barrier that prevents micelle coagulation and leads to aggregation by van der Waals interactions [30] . These results demonstrated that the pPTX/pCD nano-assembly was clearly different from pPTX micelles, showing the outstanding stability of the nano-assembly even in a large dilution and ionic concentrations similar to physiological conditions. Figure 3: Stability study of the pPTX/pCD nano-assembly and pPTX micelle. ( a ) Illustration of the dissociation of the pPTX/pCD complex in the presence of free CD. ( b ) The change in hydrodynamic radius distribution of the pPTX/pCD complex by adding 50 equivalent free CD. ( c ) The hydrodynamic radius profiles of pPTX/pCD during incubation with various equivalents free CD. ( d ) Illustration of pPTX micelle disruption by dilution or NaCl addition. ( e ) The effect of [PTX] concentration (based on the amount of PTX in pPTX) on the size of the pPTX/pCD and the pPTX micelle, as [PTX] increases from 0.03 to 0.5 mM. ( f ) The salt effect on the size of pPTX/pCD and pPTX micelle, where [PTX]=0.125 mM, [NaCl]=0, 0.1, 0.2 and 1.0 M. Error bars represent ±s.d. from n =3. Full size image The enhancement of PTX solubility in water, as seen in the high PTX loading in the polymeric nano-assembly, is critical for achieving a useful therapeutic effect. The relative water solubility of PTX in the various formulations was compared using measurements of light transmittance. Above a concentration of 10 μM, unformulated PTX was turbid with a low transmittance value, while the pPTX/pCD nano-assembly and the pPTX micelles were almost transparent, with a transmittance value greater than 80% ( Fig. 4a,b ). Due to the hydrophilic carboxylic acid groups on the polymeric backbone, the solubility of PTX in both the pPTX and the pPTX/pCD nano-assembly was drastically increased. This enhanced water solubility of the pPTX/pCD nano-assembly was also proved by the solubility-based PTX release test, which is mainly governed by the hydrolysis of ester bonds ( Supplementary Fig. 5 ). Thus, it might be advantageous to use either pPTX/pCD or pPTX to solubilize PTX, instead of the Cremophor EL–ethanol mixture used clinically for solubilizing PTX. 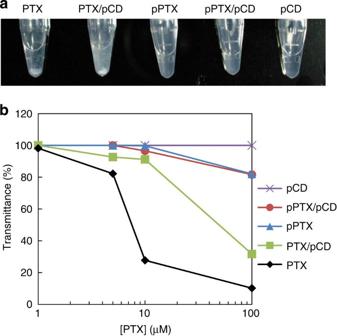Figure 4: Solubility test. (a) Optical images of solution turbidity of free PTX, PTX/pCD, pPTX, pPTX/pCD and pCD in DI water, where [PTX]=100 μM. (b) Transmittance (% T) versus the concentration for the solution of free PTX, PTX/pCD, pPTX, pPTX/pCD and pCD in DI water. Figure 4: Solubility test. ( a ) Optical images of solution turbidity of free PTX, PTX/pCD, pPTX, pPTX/pCD and pCD in DI water, where [PTX]=100 μM. ( b ) Transmittance (% T) versus the concentration for the solution of free PTX, PTX/pCD, pPTX, pPTX/pCD and pCD in DI water. Full size image Molecular dynamic simulation To further validate the stability of the pPTX/pCD nano-assembly, we conducted molecular dynamic (MD) simulations of three complexes (PTX/CD, PTX/pCD and pPTX/pCD) by employing the coarse-graining methodology in conjunction with the Martini force field ( Fig. 5 ) [31] . With the simplified model, we intend to gain qualitative insights into the stability gained by polymerization. The structures of the complexes were first modelled by allowing each complexing pair to self-assemble through 40-ns simulations with an added bias potential that favours the inclusion complex formation. ( Supplementary Figs 6,7 and Supplementary Data 1 ) The relative stabilities of these complexes were then assessed with subsequent 100-ns simulations for 10 independent trajectories towards varying concentration conditions with different box sizes, by adopting the reasonably physical Martini force field model without any biasing potential ( Supplementary Fig. 8 ). As shown in Fig. 5a , the PTX/CD complex exhibited the lowest stability on average compared with PTX/pCD and pPTX/pCD, with the smallest amount of lasting complexation at 100 ns. On average, more than 90% of monomeric PTX/CD complexes dissociated after 100 ns, whereas PTX/pCD and pPTX/pCD displayed only 20–30% PTX/CD pair dissociations after the same time. These data support the conclusion that the stability of the nano-assembly results from the multiplicity of the PTX/CD inclusion complexes formed between the two polymer conjugates [32] , [33] . 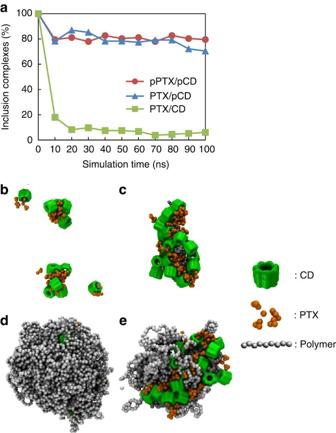Figure 5: Molecular simulation of inclusion complexes between CD and PTX. (a) Percentage of inclusion complexes between CD and PTX. (b–e) Molecular modelling structures of PTX/CD (b), PTX/pCD (c), full particle of pPTX/pCD (d) and inside view of particle of pPTX/pCD (e) after 100 ns simulations. Figure 5: Molecular simulation of inclusion complexes between CD and PTX. ( a ) Percentage of inclusion complexes between CD and PTX. ( b – e ) Molecular modelling structures of PTX/CD ( b ), PTX/pCD ( c ), full particle of pPTX/pCD ( d ) and inside view of particle of pPTX/pCD ( e ) after 100 ns simulations. Full size image Of course, our simulations do not guarantee that the relative stabilities will follow the same pattern at much longer timescales. However, within this timescale limitation, it is encouraging that the simulations present good accord with experimental findings. Based on this encouraging nature, we can further gain insight about the structural aspect that may explain the stability of the pPTX/pCD complex compared with that of the PTX/CD complex. The relatively lower stability of the PTX/CD complex could be due to the solvent exposure of hydrophobic PTXs, forcing PTX to form local aggregates ( Fig. 5b ). This could lead to the observed dissociation of the inclusion complexes. In the case of PTX/pCD, the presence of closely packed CD groups and polymer chains creates several amphipathic pockets that can accommodate free PTX molecules ( Fig. 5c ). Further, the close proximity of CD molecules allows interaction between adjacent PTX molecules that are involved in inclusion complexes, which adds stability to the complex. In fact, when one PTX/CD inclusion complex pair dissociates, the entropic gain will always be larger when the unit is free in solution than when the unit is attached to a polymer chain. Thus, thermodynamically, we can naturally expect that the binding will be stronger with polymerization. In short, the greater stability of pPTX/pCD stems from the burial of hydrophobic PTX groups combined with the entropic advantage, similar to PTX/pCD complexes. In addition, one pPTX/pCD unit contains four large amphipathic polymer chains. These polymers were found to encapsulate the PTX/CD complexes, which render the PTX groups inaccessible to solvent ( Fig. 5d,e ). In vitro anticancer effect The pPTX/pCD nano-assembly with high stability, solubility and larger PTX release rate might improve the therapeutic effect of PTX. To investigate the potential therapeutic effect of the pPTX/pCD nano-assembly, we performed cancer cell toxicity experiments using MTT assay against three cell lines: breast carcinoma MCF-7, cervical carcinoma HeLa and colorectal adenocarcinoma HCT-8. No significant toxicity was observed with the pCD and poly(MVE- alt -MAnh) polymer itself, while a dose-dependent cytotoxicity was observed with all the PTX-formulated carriers, as shown in Fig. 6a–c ; pPTX/pCD, pPTX and PTX/pCD each exhibited a higher cytotoxicity than free PTX in the three cell lines. In MCF-7 cells, an IC 50 value of pPTX/pCD was 0.08 μg ml −1 , which was about 120-fold lower than that of free PTX (9.74 μg ml −1 ). In comparison, PTX/pCD and pPTX had IC 50 values of 8.45 μg ml −1 and 0.39 μg ml −1 , respectively, which were higher than that for pPTX/pCD. IC 50 values for the pPTX/pCD were 6.62 ng ml −1 and 7.84 ng ml −1 in HeLa and HCT-8 cells; these values were less than those of free PTX (40.52 ng ml −1 and 43.35 ng ml −1 , respectively) ( Table 1 ). Importantly, pPTX/pCD exhibited the highest cytotoxicity towards all three cell lines, which was attributed to its high aqueous solubility, readily degradable ester bonds and the resultant enhanced release rate of PTX. In addition, to confirm whether cell toxicity was initiated from PTX-induced apoptosis, fluorescence-activated cell sorting (FACS) analysis was carried out in three cell lines ( Supplementary Fig. 9 ). A higher amount of apoptosis was observed in the pPTX/pCD-treated group compared with that of the PTX-treated group, indicating that PTX released from pPTX/pCD is the main reason for higher cytotoxicity. However, it is hard to ascribe the actual factor that imparts extreme stability to the pPTX/pCD nano-assembly in extracellular conditions, but the pPTX/pCD complex resulted in high cytotoxic efficacy in the cells. We presume that in extracellular conditions, the structural integrity of the nano-assembly is maintained as the partial hydrolysis remains confined mostly to the surface of the nano-assembly due to the highly entangled and condensed structure of the core domain ( Fig. 5d,e ). Once it enters the cells, the degradation of the nano-assembly may be accelerated by enzymes like esterase, resulting in the release of a large amount of free PTX in the intracellular region. 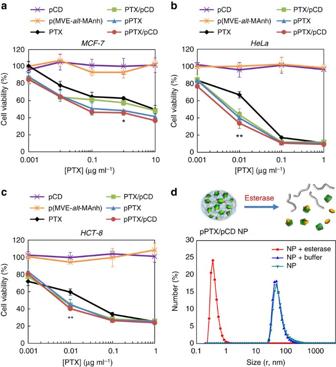Figure 6:In vitroantitumour effect of carriers. (a–c) Cell viability treated with various concentrations of PTX in PTX/pCD, pPTX and pPTX/pCD. pCD and p(MVE-alt-MAnh), which have no PTX, and free PTX were used as controls. Cells were exposed to PTX solution for 48 h. Cell viability was examined by MTT assay and normalized against the untreated cells. (a) MCF-7, (b) HeLa and (c) HCT-8 cell lines. Error bars represent ±s.d. fromn=3. Statistical analysis was done using the Studentt-test. The symbol indicates statistical significance of pPTX/pCD compared with PTX (*P<0.05; **P<0.01). (d) Enzymatic degradation of pPTX/pCD; [PTX]=60 μM; esterase from porcine liver (10 units ml−1); incubation for 10 min at 25 °C in DPBS (pH 7.4). Figure 6: In vitro antitumour effect of carriers. ( a – c ) Cell viability treated with various concentrations of PTX in PTX/pCD, pPTX and pPTX/pCD. pCD and p(MVE- alt -MAnh), which have no PTX, and free PTX were used as controls. Cells were exposed to PTX solution for 48 h. Cell viability was examined by MTT assay and normalized against the untreated cells. ( a ) MCF-7, ( b ) HeLa and ( c ) HCT-8 cell lines. Error bars represent ±s.d. from n =3. Statistical analysis was done using the Student t -test. The symbol indicates statistical significance of pPTX/pCD compared with PTX (* P <0.05; ** P <0.01). ( d ) Enzymatic degradation of pPTX/pCD; [PTX]=60 μM; esterase from porcine liver (10 units ml −1 ); incubation for 10 min at 25 °C in DPBS (pH 7.4). Full size image Table 1 Summarized IC 50 value in in vitro cytotoxicity assay. Full size table To affirm our assumption of this enzyme-triggered disintegration of the nano-assembly, we investigated the effect of an esterase on the size of the pPTX/pCD nano-assembly ( Fig. 6d ). In the presence of an esterase, the size of the nano-assembly dramatically decreased to less than 1 nm within 10 min, which suggested the esterase-mediated rapid hydrolysis of the ester linkages in the nano-assembly, leading to the disintegration of all components (CDs, PTXs and polymers) into the active constituent particles. To ascertain the role of the enzyme in triggering such disintegration, esterase was denatured by heating at 50 °C for 30 min prior to the treatment. As postulated, no such decrease in size was observed on employing denatured esterase, and large aggregates were formed instead ( Fig. 6d and Supplementary Fig. 10a ). In addition, the size of the nano-assembly was not changed when incubated with blood plasma, implying that the pPTX/pCD nano-assembly remains stable during blood circulation ( Supplementary Fig. 10b and c ). Therefore, we reiterate that the developed pPTX/pCD nano-assembly not only imparted stability to the delivery vehicle but also enabled an opportune and efficient release of PTX. The improved stability and stimuli-responsive degradation of the nano-assembly are of paramount importance in eliciting minimal side effects and maximizing therapeutic efficacy. In vivo antitumour effect Prior to the examination of in vivo antitumour activity, the biocompatibility of the carriers was investigated with a hemolysis assay. As shown in Fig. 7a , the carriers had no hemolytic effect on erythrocytes even at a high concentration of 40 μg PTX. In contrast, Taxol, the most commonly used agent in chemotherapy, showed >40% hemolytic effects under all conditions. The results indicate that Cremophor EL used for PTX solubilization is very toxic, while polymeric carriers based on hydrophilic polymers and host–guest interactions are favourable for in vivo application. 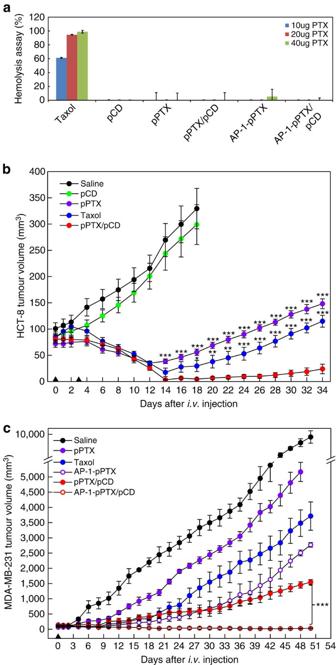Figure 7:In vivotumour-bearing mice experiments. (a) Hemolysis rates of pCD, Taxol, pPTX, AP-1-pPTX, pPTX/pCD and AP-1-pPTX/pCD under various concentrations. Error bars represent±s.d. fromn=3. (b) HCT-8 tumour growth profile treated with pPTX/pCD, pPTX, Taxol, saline and pCD. Arrows indicate tail vein injections on day 0 and 3. Error bars represent ±s.d. fromn=8. (c) MDA-MB-231 tumour growth profile treated with Taxol, pPTX, AP-1-pPTX, pPTX/pCD, AP-1-pPTX/pCD and saline. Error bars represent ±s.d. fromn=7. Statistical analysis was done using analysis of variance compared with the pPTX/pCD nano-assembly (*P<0.05; **P<0.01; ***P<0.001). Figure 7: In vivo tumour-bearing mice experiments. ( a ) Hemolysis rates of pCD, Taxol, pPTX, AP-1-pPTX, pPTX/pCD and AP-1-pPTX/pCD under various concentrations. Error bars represent±s.d. from n =3. ( b ) HCT-8 tumour growth profile treated with pPTX/pCD, pPTX, Taxol, saline and pCD. Arrows indicate tail vein injections on day 0 and 3. Error bars represent ±s.d. from n =8. ( c ) MDA-MB-231 tumour growth profile treated with Taxol, pPTX, AP-1-pPTX, pPTX/pCD, AP-1-pPTX/pCD and saline. Error bars represent ±s.d. from n =7. Statistical analysis was done using analysis of variance compared with the pPTX/pCD nano-assembly (* P <0.05; ** P <0.01; *** P <0.001). Full size image We next examined the antitumour activity of the pPTX/pCD nano-assembly using the HCT-8 xenograft mouse model. Taxol, pPTX, pPTX/pCD, pCD and saline solution were administered intravenously (twice on days 7 and 10 after tumour inoculation). The saline control and pCD groups exhibited a rapid increase in tumour size, ~300–400 mm 3 at day 25. On the other hand, Taxol and pPTX were able to suppress tumour growth in mice until day 20, but tumour regrowth was observed afterwards. Notably, mice treated with the pPTX/pCD nano-assembly showed a significant decrease in tumour progression, with the tumour almost completely disappearing, resulting in an extended survival rate ( Fig. 7b and Supplementary Fig. 11 ). The TUNEL assay was carried out to determine whether Taxol, pPTX and pPTX/pCD induced apoptosis. By observing increased apoptotic cells in the PTX-containing drug formulations, we confirmed that significant tumour inhibition observed in mice treated with Taxol, pPTX and pPTX/pCD might arise from apoptosis ( Supplementary Fig. 12 ). In addition, a relatively lower change in body weight was observed in mice treated with pPTX and pPTX/pCD, indicating that the nonspecific toxicity of pPTX and pPTX/pCD was considerably lower than that of Taxol ( Supplementary Fig. 13 ). Overall, the pPTX/pCD nano-assembly demonstrated long-term suppression of tumour growth compared with Taxol and pPTX micelles. This high antitumour efficacy of the pPTX/pCD nano-assembly might be due to less nonspecific toxicity, in vivo stability and sustained drug release induced by multivalent interaction. Although the pPTX/pCD nano-assembly showed a significant in vitro and in vivo antitumour effect against human colon cancer cells (HCT-8), it is difficult to obtain higher antitumour effect against invasive and metastatic human breast cancer cells, such as MDA-MB-231 cells, which are insensitive to PTX-induced apoptosis [34] . To surmount this problem, we functionalized the carrier system with a targeting ligand, AP-1 peptide, which has been known to target the interleukin-4 (IL-4) receptor that is overexpressed on the surface of MDA-MB-231 cells [35] , [36] , [37] . Similar to previous tumour inhibition experiments, we investigated the antitumour effect of the AP-1-conjugated nano-assembly against MDA-MB-231 cells. As shown in Fig. 7c , the pPTX micelle, which has an antitumour effect in HCT-8 cells, did not inhibit tumour growth in metastatic MDA-MB-231 cells. Taxol showed an antitumour effect in early stage until day 10, but tumour regrowth was observed afterwards. This might be due to the fast elimination of Taxol from the blood. The non-targeted pPTX/pCD nano-assembly, which was efficient in tumour growth inhibition activity in HCT-8 cells, showed moderate sustained tumour suppression in the MDA-MB-231 cell line. Compared with the non-targeted nano-assembly, the AP-1-pPTX/pCD nano-assembly showed very efficient tumour suppression in a sustained manner, and tumour regrowth was not observed until day 50, indicating the efficient and target-specific internalization of the nano-assembly into the tumour cells ( Fig. 7c and Supplementary Fig. 14 ). AP-1-pPTX micelles showed an antitumour effect until day 20, but after that the average tumour volume increased rapidly. This result suggests that AP-1-pPTX efficiently inhibited tumour growth at the early stage due to targeting and fast drug release, but sustained tumour inhibition was not obtainable due to the instability of pPTX micelles and subsequent elimination from the body. Overall, it is evident from these results that the AP-1-pPTX/pCD nano-assembly successfully inhibited tumour growth due to its high and efficient cellular uptake induced by receptor-mediated targeting and showed a long-term antitumour effect owing to its high stability in the blood through multivalent interactions. To investigate the specific interaction between the AP-1 ligand of carriers and the IL-4 receptor of cell surfaces, in vivo biodistribution of AP-1-pPTX/pCD was studied. In a single xenograft tumour model using an AP-1-negative MCF-7 cell line or an AP-1-positive MBA-MB-231 cell line, FCR-675-labelled AP-1-pPTX/pCD was systemically injected and its biodistribution was evaluated using the IVIS Spectrum system (Caliper Lifesciences, Hopkinton, MA, USA). As shown in Fig. 8a , high tumour accumulation of the carrier was observed in AP-1-positive MDA-MB-231 cell lines compared with the AP-1-negative cell line. In the dual tumour model having both an AP-1-positive MDA-MB-231 tumour and an AP-1-negative MCF-7 tumour, higher tumour accumulation of the AP-1-pPTX/pCD nano-assembly was found for the AP-1-positive tumour (right) compared with the AP-1-negative tumour (left) ( Fig. 8a ). To quantitatively investigate the accumulation of the nano-assembly in various organs, FCR-labelled AP-1-pPTX/pCD was intravenously injected and ex vivo analysis was carried out by measuring the fluorescence intensity of each organ ( Fig. 8b and Supplementary Fig. 15 ). As shown in Fig. 8c , the accumulation of AP-1-pPTX/pCD was 3.7 times higher for the AP-1-positive MDA-MB-231 tumour than for the AP-1-negative MCF-7 tumour, while a lower amount of AP-1-pPTX/pCD accumulated in the liver, kidney and gastrointestinal tract (GI) of MDA-MB-231-bearing mice compared with MCF-7-bearing mice. This result suggests that conjugation of the AP-1 peptide to the pPTX/pCD nano-assembly enhanced targeting efficiency but reduced nonspecific organ accumulation, meaning that the nano-assembly can reduce nonspecific toxicity. These results clearly indicate that the AP-1-peptide-conjugated pPTX/pCD nano-assembly can be actively accumulated and effectively taken by the AP-positive cell lines through specific interactions of AP-1 and the IL-4 receptor. 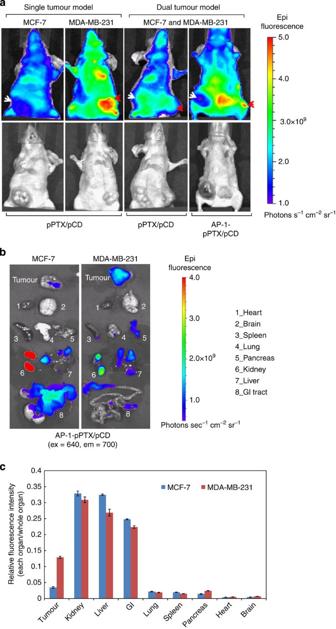Figure 8:In vivoandex vivobiodistribution. (a)In vivobiodistribution profile of MCF-7 tumour (white arrow, AP-1-negative) or MBD-MB-231 tumour (red arrow, AP-1-positive)-bearing mice treated intravenously with pPTX/pCD or AP-1-pPTX/pCD. (b)Ex vivoimages of organs retrieved from tumour-bearing mice after intravenous injection of FCR-labelled AP-1-pPTX/pCD. (c) Quantitative analysis of relative organ accumulation in each single tumour model system. Error bars represent ±s.d. analysed by IVIS spectrum small-animalin vivoimaging system. Figure 8: In vivo and ex vivo biodistribution. ( a ) In vivo biodistribution profile of MCF-7 tumour (white arrow, AP-1-negative) or MBD-MB-231 tumour (red arrow, AP-1-positive)-bearing mice treated intravenously with pPTX/pCD or AP-1-pPTX/pCD. ( b ) Ex vivo images of organs retrieved from tumour-bearing mice after intravenous injection of FCR-labelled AP-1-pPTX/pCD. ( c ) Quantitative analysis of relative organ accumulation in each single tumour model system. Error bars represent ±s.d. analysed by IVIS spectrum small-animal in vivo imaging system. Full size image Finally, we investigated the possibility for renal excretion by using IVIS. As shown in Supplementary Fig. 16 , the AP-1-pPTX/pCD complex could be excreted into the bladder, providing preliminary proof of body clearance of the nano-assembly. The clinical applications of the most effective anticancer drugs have been hampered by their extremely poor water solubility and indiscriminate distribution in the body. The use of nanocarriers has alleviated these problems to some extent by improving their aqueous stability and their preferential accumulation within the tumour via the EPR effect while minimizing toxicity. However, simple accumulation of drug-loaded nanocarriers at the tumour site does not necessarily ensure the delivery of drugs into the tumour cells. To increase cellular uptake, the nanocarriers may need to be modified with targeting ligands. In addition, drug-loaded nanocarriers should also maintain in vivo stability while circulating and be able to release their payload after being taken up by the cells. Thus, the development of rationally designed nanocarriers to realize more effective therapy is essential. In the present study, we developed a novel pPTX/pCD system that has different characteristics from other comparable NP systems for drug delivery, such as NK012 (ref. 38 ) and CRLX-101 (refs 39 , 40 , 41 ). NK012 is a micelle comprising block copolymer linked by SN-38 via ester bonds, and CRLX-101 is a self-assembled NP formed by inter- and intra-inclusion complexes comprising polymer (PEG), host (CD) and guest (camptothecin). The pPTX/pCD system was designed to encompass advantages of the above systems. The ester bonds of each CD and PTX with corresponding poly(MAnh)s were easily formed and could provide biodegradable characteristics. In addition, the host–guest interaction using two different polymers (pCD and pPTX) was employed to easily make a nano-assembly with various host–guest ratios. We envisaged that a nano-assembly fabricated using pCD and pPTX through spontaneous inclusion complexation could improve stability because of the multivalent interactions compared with the monovalent PTX/CD complex. This assumption was supported by the molecular simulation study, which indicated that the nano-assembly maintained its structural integrity while the monovalent PTX/CD complex dissociated easily. In addition, hydrophilic polymers were found to be exposed and covered on the surface of the nano-assembly and thereby encapsulated the PTX/CD complex segments into the core, which consequently protects them from nonspecific enzymatic degradation from esterase during blood circulation. The experimental studies also showed that the K a value of the nano-assembly was 10 4 -fold higher than the monovalent complex. This high stability of the nano-assembly may increase its circulation time in the blood and prevent the premature release of drugs, thereby minimizing toxicity to normal tissue. The prolonged circulation might also increase the possibility of the nano-assembly reaching the tumour site. To examine whether our nano-assembly can effectively target aggressive and metastatic cancer cells, we established an MDA-MB-231 xenograft mouse model. Noticeably, the AP-1-conjugated nano-assembly demonstrated significant tumour inhibition compared with the non-targeted nano-assembly. This high in vivo antitumour efficacy of the AP-1-conjugated nano-assembly might be explained by the combination of enhanced accumulation at the tumour site (EPR effect), followed by effective cellular uptake (receptor-mediated endocytosis). Although intensive further studies to warrant a complete kidney clearance are required, given the enhanced stability, stimuli-responsive drug release and effective tumour targeting through passive and active targeting mechanisms, an AP-1-conjugated nano-assembly shows promising potential as a drug-delivery system for cancer therapy. Conjugation of β-CD and PTX to poly(MAnh)s Prior to the reaction, β-CD was dried in a vacuum oven at 110 °C for 12 h to remove the water content. Next, 1 g of β-CD was dissolved in dried DMF (20 ml) under nitrogen, and 7.0 mg of LiH was added as a powder into the CD solution. In order to avoid linking more than one hydroxyl group of CD and the polymer backbone, only one hydroxyl group on the CD molecule was selectively deprotected by using LiH in a stoichiometric ratio with CD [41] , [42] , [43] , [44] . The solution was stirred for 12 h at 25 °C. A solution of 90 mg poly(IB- alt -MAnh) dissolved in 10 ml anhydrous DMF was dropped into the activated CD solution and then stirred at 25 °C. After 12 h, DMF was evaporated under vacuum, and the residual solid was dissolved in 5 ml deionized (DI) water. To remove unreacted CDs and other byproducts, the resultant product was dialyzed in a dialysis membrane (MWCO 3500) with DI water for 48 h and lyophilized. The final product, poly(IB- alt -MAnh)- graft -CD x (pCD x ), was obtained as a white solid. Next, 33.3 mg of PTX was dissolved in dried DMF (5 ml) under nitrogen, and 1.0 mg of LiH was added as a powder into the PTX solution. The 2′-hydroxyl group of PTX is more reactive than the 1- and 7-hydroxyl groups owing to less steric hindrance, and therefore this 2′-hydroxyl group of PTX preferentially reacts with the anhydride groups of the MVE copolymer. The solution was stirred for 12 h at 25 °C. A solution of 156 mg poly(MVE- alt -MAnh) dissolved in 10 ml anhydrous DMF was dropped into the activated PTX solution and then stirred at 25 °C. After 12 h, the DMF was evaporated under vacuum and the residual solid was dissolved in 2 ml of DI water. The reaction was monitored by TLC (silica plate; eluent, CHCl 3 :MeOH [10:1]; R f [PTX]=0.7; R f [conjugate]=0). To remove unreacted PTXs and other byproducts, the resultant product was dialyzed in a dialysis membrane (MWCO 3500) with DI water for 48 h and lyophilized. The final product, poly(MVE- alt -MAnh)- graft -PTX y (pPTX y ), was obtained as a pink solid. Formation of the pPTX/pCD nano-assembly Two polymer conjugates, pCD 20 and pPTX 7 (molar ratio of PTX/CD=1), were dissolved in 20% (v/v) ethanol solution to obtain a 0.1% (w/v) PTX solution. This solution was stirred for 12 h at 25 °C and then lyophilized. The resultant powder was dissolved in DI water to make 2 mM of PTX stock solution. The drug encapsulation (loading) efficiency of PTX was calculated by measuring the weight % of PTX in the pPTX/pCD nano-assembly and was found to be 5.1%. As controls, PTX/pCD 20 and pPTX 7 were formulated using a similar method. In the case of PTX/pCD 20 , free PTX was used instead of pPTX 7 . For pPTX 7 , no CD molecules were added during the formulation process. Measurement of hydrodynamic size and zeta potential The hydrodynamic sizes of various samples (pPTX/pCD, pPTX, PTX/pCD, free PTX and pCD) were measured by DLS using a Zetasizer Nano S DLS system (Malvern Instruments, Malvern, UK). The surface charges were measured by determining the zeta potential using a Zetasizer Nano Z potential analyzer (Malvern Instruments). The final PTX concentration of the nano-assembly solution was adjusted to 125 μM in DI water ( n =3). In addition, the influence of concentration of PTX on the size of pPTX/pCD and pPTX was determined by DLS, using PTX solutions between 0 mM and 0.5 mM. The effect of NaCl (0 M–1.0 M) on pPTX/pCD and pPTX (125 μM PTX) was evaluated by DLS. TEM analysis The morphologies of pPTX/pCD, pPTX and PTX/pCD were examined by TEM. First, 1 μl of the solutions (125 μM PTX) was transferred onto hydrophilic-treated grids, and the grids were left overnight to dry completely. Then, samples were imaged by TEM (HITACHI-7066, Japan) operating at 80 kV acceleration voltages without any staining. Disintegration of pPTX/pCD NPs by free CD molecules To verify that pPTX/pCD NP formation was triggered by host–guest inclusion complexation of CD and PTX, DLS measurement was carried out. A pPTX/pCD NP solution was prepared. We added 0, 1, 10 and 50 equivalent of free CD to this solution and incubated it at room temperature for 12 h. Next, the changes in the hydrodynamic size of the NPs were measured after 1, 3, and 12 h of incubation ( n =3). Determination of the association constant To determine the association constants of the pPTX/pCD NP, we used competition between the pPTX and the fluorescent probe TNS. TNS is a fluorescent guest molecule that shows negligible fluorescence in aqueous solutions but exhibits strong fluorescence when included in the hydrophobic cavity of CD, forming a TNS/CD complex. The increased amounts of CD to aqueous TNS solution enhanced fluorescence intensity. In the presence of PTXs, which were competitive molecules to TNS, fluorescence of the TNS/CD solution was reduced. We calculated the K a of PTX/CD by determining the slope of the double reciprocal plots from the two data sets. One calculation was done for TNS/CD and the other one was done for the mixture of TNS/CD and PTX/CD. Using a similar method, the K a of the pPTX/pCD NP was measured using pCD and pPTX instead of free CD and free PTX. The fluorescence of the TNS solution in the presence of pCD and pPTX was measured using a fluorescence spectrophotometer (RF-5301PC, Shimadzu, Japan). The excitation wavelength was 320 nm, while the emission wavelength was from 400–600 nm. Uncorrected fluorescence values were converted into relative fluorescence, using F rel = I obs / I 0 , where I 0 is the fluorescence intensity at [pCD]=0. First, the fluorescence intensity enhancement of TNS (10 μM) was observed as an increasing concentration of pCD ([CD]=10 μM–100 μM). Second, the same experiment was conducted using pPTX ([PTX]=10 μM) as a competitor to TNS. The association constants of pPTX/pCD were determined in this indirect method by monitoring the attenuation of the TNS fluorescence intensity. Double reciprocal plots of the data from the first titration (with guest TNS) and from the second titration (with guest TNS and competitive guest pPTX) were drawn. The dissociation constant K i can be formulated as follows equation (1) [28] : where K i is the dissociation constant for the pPTX; K 1 is the negative x intercept of the first curve (association constant for TNS); K 2 is the negative x intercept of the second curve; and [I] is the pPTX concentration. Thus, the association constant of pPTX/pCD was calculated using 1/ K i . As a control, the association constants of PTX/CD, PTX/pCD, and pPTX/CD were measured following the same procedure. Molecular dynamic simulations of the pPTX/pCD nano-assembly Three-dimensional structures of the complexes were first modelled by 50–100 ns self-assembly simulations with an added bias potential that favours the inclusion complexation. We then tried to assess the stabilities of these complexes with additional 100 ns simulations by adopting only the reasonably physical Martini force field model with the biasing potential completely turned off. The detailed experimental procedures are described in the Supplementary Methods and Supplementary Data 1 . Analysis of transmittances To compare the water solubility of PTX formulated in pPTX/pCD with that of free PTX, we observed their optical transmittance by varying the concentration of PTX (0 μM–100 μM PTX). Transmittance at 500 nm was measured using an ultraviolet-visible spectrometer (UV2550, Shimadzu, Japan). pCD, pPTX, and PTX/pCD were used as controls. In vitro cytotoxic assay The cytotoxicity of the various PTX formulations, which were free PTX, PTX/pCD, pPTX and pPTX/pCD, and the PTX-free polymer conjugates, pCD and poly(MVE- alt -MAnh), were estimated using an MTT assay. MCF-7 (human breast carcinoma cells, KCLB30022), HeLa (human cervical carcinoma cell, KCLB10002) and HCT-8 (human colorectaladenocarcinoma cell, KCLB10244) were obtained from the Korea Cell Line Bank (KCLB). MCF-7 (or HeLa, HCT-8) cells were seeded in 96-well plates at a density of 5 × 10 3 cells per well and incubated for 24 h. Various concentrations of samples (all performed at equivalent PTX concentrations of 0.001, 0.01, 0.1, 1, and 10 μg ml −1 ) were treated in 200 μl of culture medium. Cells were then incubated for 48 h, and the media were replaced with 200 μl of fresh medium with 20 μl of 5 mg ml −1 MTT solution. After 4 h of incubation, the medium was removed and 150 μl of DMSO was added to each well to dissolve the internalized purple formazan crystals. An aliquot of 100 μl was taken from each well and transferred into a fresh 96-well plate. The absorption was measured at 570 nm using a microplate spectrofluorometer (VICTOR3 V_Multilabel Counter; Perkin Elmer, Wellesley, MA, USA). The relative percentage of the control (untreated) cells, which were not exposed to the transfection system, was used to represent 100% cell viability. All results are expressed as mean±s.d. Statistical analysis was done using Student t -tests with a 95% confidence interval as the threshold for significance. Enzymatic degradation of pPTX/pCD nano-assembly The pPTX/pCD nano-assembly ([PTX]=60 μM) was dispersed in DPBS (pH 7.4). To induce enzymatic degradation of NPs, a solution of esterase from porcine liver (10 units ml −1 , 500 μl, e code 3.1.1.1, Sigma) was added to the 500 μl of NP solution and incubated at 25 °C for 10 min. For a control experiment, denatured esterase was prepared by heating at 50 °C for 30 min before addition to the NP solution. The hydrodynamic sizes of samples were measured by DLS. Synthesis of FCR-AP-1-conjugated pPTX/pCD First, FCR-675 dye (Bioacts, Korea) and AP-1 peptide were conjugated to pPTX through an amine-anhydride reaction and a (2-pyridyldithio)-ethylamine linker, respectively. The conjugation ratio of FCR-675 to pPTX was confirmed by quantitative fluorescence at 675 nm excitation and 692 nm emission. AP-1 conjugation efficiency was ascertained from the quantitative UV absorbance of released 2-pyridinethione at 370 nm by the thiol exchange reaction between the (2-pyridyldithio)-ethylamine linker and DTT. Subsequently, pPTX- graft -FCR/AP-1 was complexed with pCD (mole ratio of PTX/CD=1) to obtain the FCR-AP-1-conjugated pPTX/pCD nano-assembly. The detailed synthetic procedure is illustrated in the Methods section of Supplementary Information . Hemolysis assay Hemolysis studies were carried out for pCD, Taxol, pPTX micelles, pPTX/pCD, AP-1-pPTX micelles and AP-1-pPTX/pCD according to a previous report [45] . The release of haemoglobin from the erythrocytes was used for toxicity measurements of these carriers. Fresh mouse blood was collected into a 0.5 ml EDTA tube. The volume of the blood sample was diluted 10 times with PBS and centrifuged at 2,000 r.p.m. for 15 min. The supernatant was decanted, and the precipitate was rinsed three times with PBS, followed by centrifugation at 2,000 r.p.m. for 15 min. The concentration of resulting blood cells was adjusted to 2% (v/v). Sample solutions (20 μl) were mixed with 200 μl blood cells, and the resulting suspensions were incubated at 37 °C for 3 h. The samples were then centrifuged at 2,000 r.p.m. for 15 min. The absorbance of the supernatant was measured at 541 nm to determine the amount of haemoglobin release. Zero hemolysis and 100% hemolysis consisted of red blood cells suspended in physiological saline and distilled water, respectively. The percentage of hemolysis was determined as follows equation (2): where A sample is the absorbance of the sample, A 100 is the absorbance of completely lysed red blood cells in distilled water, and A 0 is the absorbance of zero hemolysis. All hemolysis assays were done in triplicate. Statistical analysis of the hemolytic activity of different polymer compositions was done using Student t -tests with a 95% confidence interval as the threshold for significance. In vivo animal experiments All animal experiments were approved by the Postech Biotech Center Ethics Committee. HCT-8 cells (1 × 10 7 ) were inoculated subcutaneously into the flank of each female BALB/c- nu/nu mice (weight 18±2 g). The mice were randomly divided into five groups (eight mice per group) and treated with 100 μl of physiological saline, pCD, Taxol, pPTX micelles, pPTX/pCD nano-assembly (4 and 10 mg kg −1 PTX) on day 7 and 10 post inoculation. The antitumour effect against HCT-8 growth was assessed by measuring the diameter of the tumours with an electronic caliper every other day. Each tumour was measured in two dimensions by caliper, and the recorded measurements were converted to tumour mass using the formula for a prolate ellipsoid as follows equation (3): where a is the longer and b is the shorter dimension. The samples were injected through the tail vein. After treatment, tumour progression in the mice was monitored until tumours became too large or ulcerated, at which time the mice were killed (on day 41 post inoculation). Body weight change and survival rates were also recorded. The survival rate was calculated from day 0 from HCT-8 inoculation to the day of death (on day 41 post inoculation). Kaplane–Meier survival curves were plotted for each group. MDA-MB-231 (human breast adenocarcinoma cells, KCLB30026) cells were obtained from the Korea Cell Line Bank (KCLB). MDA-MB-231 human breast cancer cells (1 × 10 7 ) were injected subcutaneously into the flank of each female BALB/c- nu/nu mice. After the tumours had grown to ~90–120 mm 3 , mice were divided into six groups (seven mice per group). Physiological saline, Taxol, pPTX micelles, pPTX/pCD nano-assembly, AP-1-pPTX micelles and AP-1-pPTX/pCD nano-assembly (administered at a PTX equivalent dose of 20 mg kg −1 ) were injected via the tail vein into one of the six groups. After treatment, tumours were measured every day until they reached a volume of 1 × 10 4 mm 3 , at which time the mice were killed. All results are expressed as mean±s.d. One-way or two-way analysis of variance was performed to demonstrate statistical differences; survival curves and body weight curves were also calculated from the software GraphPad Prism 6 for Windows. In vivo biodistribution assay In vivo near infrared imaging was performed using an IVIS spectrum small-animal in vivo imaging system (Caliper Life Sciences). The FCR-675-labelled pPTX/pCD nano-assembly (100 μl) was injected through the tail vein of dual tumour (MCF-7 and MDA-MB-231)-bearing mice 14 days post inoculation. The FCR-675-labelled AP-1-pPTX/pCD nano-assembly (100 μl) was injected through the tail vein of each single tumour (MCF-7 and MDA-MB-231) and dual tumour-bearing mouse 14 days post inoculation. The mice were anesthetized with 1.5–2% isoflurane and placed on an animal plate and heated to 37 °C. The imaging was performed at 10 min, 1 h, 4 h, and 24 h post injection, using a Cy5.5 filter set (excitations 640 and 675 nm and emissions 700 and 720 nm). After in vivo imaging, the mice were killed and the major organs were collected for ex vivo imaging. Each organ was rinsed with PBS three times and put into the board, and the fluorescent images were detected. For each single tumour model, the raw fluorescence of each organ (images in Fig. 8b ) was recorded as an absolute value ( Supplementary Fig. 15 ). To more clearly present the targeting efficiency, bar data were converted to the relative intensity of accumulation (graph in Fig. 8c ) by calculating the ratio of corresponding intensity accumulated for each organ out of the sum of the total intensity accumulated for whole organs. How to cite this article : Namgung, R. et al. Poly-cyclodextrin and poly-paclitaxel nano-assembly for anticancer therapy. Nat. Commun. 5:3702 doi: 10.1038/ncomms4702 (2014).